General incorporation of diverse components inside metal-organic framework thin films at room temperature Porous metal-organic frameworks (MOFs) demonstrate great potential for numerous applications. Although hetero-functional components have been encapsulated within MOF crystalline particles, the uniform incorporation of functional species with different sizes, shapes and functions in MOF thin films with dual properties, especially at room temperature and without the degradation of the MOF framework, remains a significant challenge towards further enriching their functions for various purposes. Here we report a general method that can rapidly encapsulate diverse functional components, including small ions, micrometre-sized particles, inorganic nanoparticles and bioactive proteins, in MOF thin films at room temperature via a metal-hydroxide-nanostrand-assisted confinement technique. These functional component-encapsulated MOF composite thin films exhibit synergistic and size-selective catalytic, bio-electrochemical, conductive and flexible functionalities that are desirable for thin film devices, including catalytic membrane reactors, biosensors and flexible electronic devices. Metal-organic frameworks (MOFs) [1] , [2] , which are self-assembled from organic ligands and metal ions, are highly promising porous crystalline materials with the strong potential for gas separation [3] , [4] , [5] , [6] , [7] , [8] , [9] , [10] , [11] , [12] , [13] , [14] , chemical sensors [15] , [16] , [17] , [18] , catalysts [19] , [20] , [21] , [22] and optical devices [23] because of their large and accessible specific surface areas, uniform and tunable pore sizes, and diverse properties. However, to further enrich or expand the functionalization of MOFs, in an approach similar to zeolites [24] , [25] , [26] , new synergistic properties have been achieved by incorporating functional species into MOFs to form composite materials that cannot be obtained from the parent MOF counterparts [27] . The incorporation of functional components into MOFs is typically accomplished by one of three methods: the incorporation of inorganic nodes through ion exchange or in situ doping [28] , [29] ; organic ligand modification [30] , [31] or the encapsulation of functional components [27] . Currently, the encapsulation process is widely used to incorporate hetero-particles with new functions into MOFs because the former two methods are limited to covalent bonding and coordination chemistry. Solution impregnation, gas-phase infiltration and solid grinding have been applied to introduce precursors into the preformed MOF host, which is then converted to the corresponding functional components encapsulated in the MOFs [32] , [33] . However, in this two-step approach, nonselective deposition at the outer surface of the MOF host is unavoidable, and particle size and morphology are limited by the cavities of the MOF host. In addition, the framework may suffer degradation during nanoparticle formation [32] , [34] . Recently, another more attractive one-pot approach has been developed that involves the addition of preformed functional particles into the MOF precursor solution and the in situ formation of MOF-encapsulated functional particles during MOF growth [33] . However, nanoparticles (NPs) tend to dissolve or agglomerate under the acidic environment created by the dissociation of ligands during this solution process. Therefore, surface modification is required to initiate the nucleation and growth of the MOFs around the nanoparticle [27] , [35] , [36] , [37] , [38] , [39] , [40] , [41] , [42] . But, the direct nucleation of MOF crystals in the growth solution is not prevented. Afterward, to confine the growth of MOFs on the surfaces of nanoparticles, metal oxide nanostructures can be employed as a metal source that is directly converted to an MOF-surrounded composite [43] , [44] . Similarly, Falcaro et al. have applied functional nanoparticle-encapsulated α-hopeite as a nucleating agent to position and encapsulate the functional components in MOF-5 with core/shell structures [45] , [46] . However, most of the aforementioned methods require relatively high temperatures and long reaction times [27] , [34] , [38] , [39] , [40] , [41] , [42] , [43] , [44] , [45] , [46] , and the obtained NP/MOF composite powders [27] , [34] , [38] , [39] , [40] , [41] , [42] , [43] , [44] are not suitable for thin film devices [10] , [43] , [44] . Furthermore, the aforementioned nanoparticles are limited to solid inorganics and polymers that are several to hundreds of nanometres in size [27] , [33] , [34] , [35] , [36] , [37] , [38] , [39] , [40] , [41] , [42] , [43] , [44] . Hence, the direct encapsulation of ions, inorganic and organic materials as well as bioactive proteins in MOFs at room temperature, without limiting the size, shape and classification and with a short processing time, should ultimately yield functional MOF composite thin films for a wide variety of purposes [47] . Here we develop a general method for the synthesis of heterogeneous functional components (ions, inorganics, polymers, carbon nanotubes and proteins with various sizes, shapes and dimensions) encapsulated in MOF thin films with thicknesses of several micrometres, both on porous substrates and in free-standing form, through a confinement-assisted growth process at room temperature within 1–2 h. The functional components are homogenously pre-embedded into a nanofibrous metal precursor thin film by simply filtering the mixture of a solution of metal hydroxide nanostrands (MHNs) and dispersions of functional components on a porous support that can be peeled from the substrate to be free-standing. The nanofibrous MHN porous networks not only serve as the metal source but also firmly confine the functional species during MOF growth. Our recent work confirmed that MHN thin films can be rapidly converted to MOF thin films through an outside-inner growth process involving immersion in an organic ligand solution at room temperature [10] , similar to the conversion of copper hydroxide NPs to HKUST-1 crystals at room temperature [48] . The initial outer MOF layer prohibits escape of the pre-embedded functional component significantly, there is no limitation of the size, dimensions and shape, or classification of the encapsulated functional components, which can be ions, nanoparticles, polystyrene (PS) spheres with sizes ranging from less than 1 nm to several micrometres, one-dimensional single-walled carbon nanotubes (SWCNTs), bioactive proteins or micrometre-sized PS spheres. The prepared composite MOF thin films exhibit synergistic properties, including size-selective catalysis, catalyst membrane reactors, bioactive electrochemical sensors, and flexible and electric conductivity, as a result of combining the porous structures of MOFs and the functional properties of the encapsulated components. Single functional component-encapsulated MOF composite thin films Owing to the unique properties of MHNs, including isolation and good dispersion in solution, a highly charged surface, small diameter and long length, MHN mesoporous thin films are easily formed through a simple mixture and filtration process and then can be rapidly converted into MOF thin films at room temperature by immersion in an organic ligand solution [10] . In addition, negatively charged functional nanoparticles, molecules, SWCNTs and proteins have been uniformly incorporated into MHN mesoporous thin films by simply mixing the functional component dispersion with a MHN solution, followed by a filtration process [49] . Therefore, the formation of functional component-encapsulated MOF composite thin films is expected. The preparation process of particle/HKUST-1 (Cu 3 (BTC) 3 ·3H 2 O) composite thin films encapsulating [AuCl 4 ] − , Au NPs (20 nm), proteins (ferritin and glucose oxidase (GOx)), PS spheres and SWCNTs is illustrated in Fig. 1a . Briefly, copper hydroxide nanostrands (CHNs; functional component composite thin films) are formed by mixing the corresponding solutions or dispersions with a CHN solution and filtering on porous substrates ( Supplementary Fig. 1 ). The positively charged surfaces of CHNs can attract negatively charged ions ( Supplementary Fig. 1a ), Au NPs (20 nm) ( Supplementary Fig. 1b ), proteins ( Supplementary Fig. 1c ) and nitrate acid-treated SWCNTs by electrostatic interaction ( Supplementary Fig. 1i,j ). The filtration process guarantees the uniform distribution of neutral PS and positively charged Fe 3 O 4 nanoparticles (10–30 nm) in the CHN films ( Supplementary Fig. 1g,h,k and l ) because the sizes of the PS and Fe 3 O 4 nanoparticles are larger than the pore size of the CHN layer, which is approximately 10 nm (ref. 49 ). The particles should be restricted on the surface of the pre-filtered CHN thin layer during filtration. As time passes, increasingly more new CHNs are accumulated, and the particles become submerged in the final CHN networks. These results clearly demonstrate that all particles disperse very well in the CHN thin films. The prepared functional component/CHN composite thin films are reacted with 10 ml of a 5 mM H 3 BTC water/ethanol solution with a volume ratio of 1:1 at room temperature for 1 h and then are converted to the corresponding functional component-encapsulated HKUST-1 (Cu 3 (BTC) 2 ) composite thin films. We present the corresponding scanning electron microscope (SEM) images of the obtained functional component-encapsulated HKUST-1 composite thin films with [AuCl 4 ] − ions ( Fig. 1b,c ), Au NPs (20 nm; Fig. 1d,e ), ferritin ( Fig. 1f–h ), GOx ( Supplementary Fig. 2 ), 620-nm PS spheres ( Fig. 1i,j ), 1-μm PS spheres ( Supplementary Fig. 3a,b ) and SWCNT ( Fig. 1j,k ). Relatively large PS spheres and fibrous SWCNTs are clearly observed and uniformly encapsulated within the HKUST-1 crystalline thin films. Although only several PS spheres are partially located on the HKUST-1 crystal surface, most are embedded in the MOF crystals ( Fig. 1h,i ). Remarkably, surface and cross-sectional SEM images clearly demonstrate that, in the cases of [AuCl 4 ] − , Au NPs (20 nm), proteins, and SWCNTs, continuous thin films are formed with well-intergrown MOFs. The thicknesses of [AuCl 4 ] − , Au NPs (20 nm) and protein/HKUST-1 composite thin films are approximately 3 μm; the thickness of SWCNTs/HKUST-1 is approximately 4.8 μm. The corresponding X-ray diffraction (XRD) patterns of all samples ( Supplementary Fig. 4a–f ) are assigned to a HKUST-1 (refs 50 , 51 ) phase, with no additional phases present. The absence of Au peaks is due to the small number (5 wt.%) of Au NPs (20 nm), which confirms that all Au NPs are fully encapsulated within the HKUST-1 host. Transmission electron microscope (TEM) images of a single crystal from Au NP (20 nm)/HKUST-1 ( Fig. 2a and Supplementary Fig. 5 ), [AuCl 4 ] − /HKUST-1 ( Supplementary Fig. 6 ) and ferritin/HKUST-1 ( Fig. 2e ) composite thin films by mechanical grinding and sonicating clearly reveal that multiple Au NPs (20 nm) and ferritins are encapsulated in the HKUST-1 host crystals. 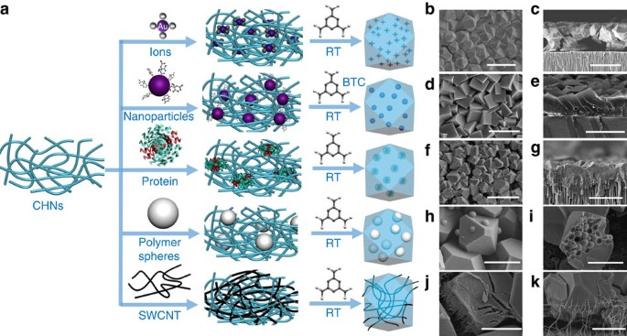Figure 1: Illustration of the synthesis process and SEM images. (a) Schematic illustration of the synthesis process of diverse functional components encapsulated HKUST-1 composite thin films through a pre-confined technique by using CHNs; (b,c) [AuCl4]−ions, (d,e) 20 nm Au nanoparticles (20 nm), (f,g) ferritin, (h,i) 620 nm PS sphere and (j,k) SWCNT, encapsulated HKUST-1 composite thin films, respectively. The scale bars are (b) 3 μm; (c) 4 μm; (d,e) 3 μm; (f) 5 μm; (g,h) 3 μm; (i) 5 μm; (j) 3 μm; (k) 2 μm, respectively. Figure 1: Illustration of the synthesis process and SEM images. ( a ) Schematic illustration of the synthesis process of diverse functional components encapsulated HKUST-1 composite thin films through a pre-confined technique by using CHNs; ( b , c ) [AuCl 4 ] − ions, ( d , e ) 20 nm Au nanoparticles (20 nm), ( f , g ) ferritin, ( h , i ) 620 nm PS sphere and ( j , k ) SWCNT, encapsulated HKUST-1 composite thin films, respectively. The scale bars are ( b ) 3 μm; ( c ) 4 μm; ( d , e ) 3 μm; ( f ) 5 μm; ( g , h ) 3 μm; ( i ) 5 μm; ( j ) 3 μm; ( k ) 2 μm, respectively. 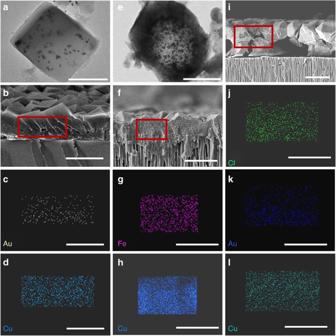Figure 2: Transmission and scanning electron microscopy and the corresponding element maps. (a–d) Au NPs (20 nm)/HKUST-1 composite thin film; (e–h) Ferritin/HKUST-1 composite thin film; (i–l) [AuCl4]−/HKUST-1 composite thin film. The scale bars are (a) 500 nm, (b) 3 μm, (c,d) 2 μm, (e) 200 nm, (f) 3 μm, (g,l) 2 μm, respectively. Full size image Figure 2: Transmission and scanning electron microscopy and the corresponding element maps. ( a – d ) Au NPs (20 nm)/HKUST-1 composite thin film; ( e – h ) Ferritin/HKUST-1 composite thin film; ( i – l ) [AuCl 4 ] − /HKUST-1 composite thin film. The scale bars are ( a ) 500 nm, ( b ) 3 μm, ( c , d ) 2 μm, ( e ) 200 nm, ( f ) 3 μm, ( g , l ) 2 μm, respectively. Full size image Energy-dispersive X-ray analysis spectroscope (EDS) mapping images recorded from the cross-sections of Au NP (20 nm), ferritin and [AuCl 4 ] − /HKUST-1 composite thin films are shown in Fig. 2c,d,f,h and j–l , respectively. Figure 2c,d , recorded from the marked area in Fig. 2b , shows that the depth distributions of Au and Cu are uniform in the Au NP (20 nm)/HKUST-1 composite thin film. Figure 2f–h , recorded from the area marked in Fig. 2e , demonstrates that Fe and Cu also homogeneously distributed throughout the entire cross-section of the ferritin/HKUST-1 composite thin film. Figure 2i–k , recorded from the area marked in Fig. 2h , shows that Au, Cl and Cu are distributed uniformly in the [AuCl 4 ] − /HKUST-1 composite thin film. The weight ratios of the copper in HKUST-1 and that in the functional components summarized from EDS spectra ( Supplementary Fig. 7 ) are shown in Supplementary Table 1 and are in consistent with those in the corresponding precursors ( Supplementary Table 1 ). These results indicate that [AuCl 4 ] − , Au NPs and ferritin are fully encapsulated in the HKUST-1 host and do not escape during HKUST-1 crystal growth. PS spheres and SWCNTs are sufficiently large to be visible in SEM images ( Fig. 1i–l ), and EDS maps were not recorded. These results confirm that all examined functional components are uniformly encapsulated within HKUST-1 crystal thin films. In an examination of zinc hydroxide nanostrands (ZHNs) in place of CHNs, an Au NP (20 nm)-encapsulated MOF-5 (zinc-related MOFs) composite thin film was also prepared through a similar process (details in the Methods section). Supplementary Fig. 8 clearly shows that Au NPs (20 nm) are uniformly incorporated into the MOF-5 matrices ( Supplementary Fig. 9 ). The general method presented here could be applied to the design of functional component-encapsulated MOF thin films. Bi-functional component-encapsulated MOF composite thin films Most previously reported functional component-encapsulated MOF composites incorporate a single functional component [27] , [34] , [38] , [39] , [40] , [41] , [42] , [43] , [44] , [45] , which limits their functionality and applications. However, by our method, two functional components, ferritin and 20-nm Au NPs, are successfully co-incorporated into HKUST-1 thin films through a one-pot process ( Fig. 3 ). Ferritin and Au NPs are pre-confined within CHN precursors by filtering a mixture suspension of ferritin, Au NPs and CHNs on a porous substrate. After reacting with 5 mM H 3 BTC water/ethanol solution with a volume ratio of 1:1 solution at room temperature for 1 h, ferritin and Au NPs are uniformly distributed in HKUST-1 matrices ( Fig. 3 ). XRD results ( Supplementary Fig. 6g ) further confirm the formation of HKUST-1, indicating that our technique is general and can introduce various components with different functions and composites into MOF thin films through a one-pot process. This technique should provide a promising preparation method for MOF thin films with multi-functions for diverse applications. 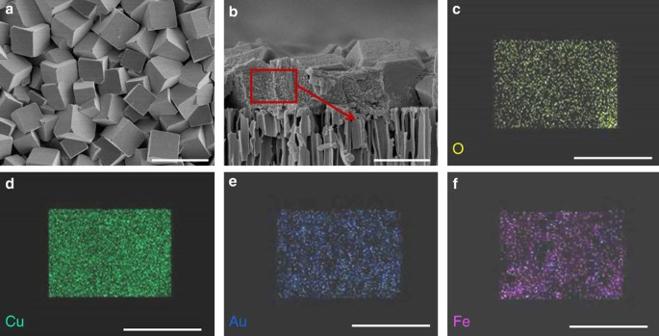Figure 3: Characterization of Au NP and ferritin HKUST-1 composite thin films. (a) Surface and (b) cross-sectional SEM images; (c–f) elements mapping images of O, Cu, Au and Fe, respectively. The scale bars are (a) 5 μm, (b) 2 μm, (c–f) 1 μm, respectively. Figure 3: Characterization of Au NP and ferritin HKUST-1 composite thin films. ( a ) Surface and ( b ) cross-sectional SEM images; ( c – f ) elements mapping images of O, Cu, Au and Fe, respectively. The scale bars are ( a ) 5 μm, ( b ) 2 μm, ( c – f ) 1 μm, respectively. Full size image Sandwiched MOF composite thin films More interestingly, sandwiched composite MOF thin films are also obtainable through a one-pot growth process. As a demonstration, two sandwich samples were synthesized. First, a CHN/PS/CHN sandwich thin film was formed by alternately filtering CHNs and PS spheres on anodic alumina oxide (AAO) substrates ( Supplementary Fig. 10a,b ). The PS sphere layer is clearly sandwiched between the two CHN layers. After reacting with 10 ml of a 5 mM H 3 BTC water/ethanol solution with a volume ratio of 1:1 at room temperature for 1 h, HKUST-1/PS/HKUST-1 sandwiched composite thin films were obtained ( Supplementary Fig. 10c ). The layer of PS spheres does not change in location and is sandwiched by HKUST-1 layers. In addition, after the addition of the obtained HKUST-1/PS/HKUST-1 composite film to N , N -dimethyl-formamide (DMF) and sonication for 15 min at room temperature, the PS spheres were fully dissolved, and ordered spherical hole arrays were produced in individual MOF crystals ( Supplementary Fig. 10d,e ). The duplicated ordered porous arrays in HKUST-1 crystals may have potential for photonic devices [52] , [53] . Similarly, a HKUST-1/SWCNTs/HKUST-1 sandwich composite thin film is also prepared, in which SWCNTs are sandwiched by CHN layers ( Supplementary Fig. 11a,b ). After reacting with H 3 BTC, the SWCNT layer is fully sandwiched by the HKUST-1 crystal layers in the final HKUST-1/SWCNT/HKUST-1 composite thin film ( Supplementary Fig. 11c ). Enzymatic performance of GOx/HKUST-1 composite thin films In the reaction between MHNs and organic ligands, water is the only by-product besides MOF formation. Furthermore, the reaction is conducted at room temperature, thus, this process is very gentle and environmental friendly. The dissociation or dissolution of functional components is avoided, allowing the incorporation of bio-components into MOFs without degrading their bio-functions. The enzymatic activity of GOx, which is very sensitive to glucose [54] , [55] , [56] , [57] , is reserved after encapsulation into HKUST-1 matrices ( Fig. 4 and Supplementary Fig. 12 ). To examine the bioactivity of incorporated GOx in HKUST-1, cyclic voltammetry (CV) data were collected for a small piece of the prepared GOx/HKUST-1 composite thin film ( Supplementary Fig. 2 ) in the presence and absence of glucose. The curves of pure HKUST-1 in the presence of glucose are similar to that of the GOx/HKUST-1 composite thin film in the absence of glucose ( Fig. 4a ). Similar CV curves are also observed on a pure glass carbon electrode (GCE; Supplementary Fig. 12a ). The reduction peaks of pure HKUST-1 and glass carbon are generated from the reduction of oxygen [54] , [55] , [56] . However, the redox current of a GOx/HKUST-1 composite thin film in the same negative potential range of −0.4 to −1.0 V dramatically decreases upon the addition of glucose, exhibiting the same effect as that of pure GOx immobilized on a GCE ( Supplementary Fig. 12b ). The competitive reactions of oxygen and glucose oxidation through the direct electron transfer of GOx can reduce the oxygen reduction current and have been used for glucose sensing [55] , [56] . The decrement of the reduction current of the GOx/HKUST-1 electrode in the presence of glucose should be due to encapsulated GOx. The relationship between the current and glucose concentration is shown in Fig. 4b . Glucose (0.1 mM, 20 μl) was added to a 20-ml phosphate-buffered saline (PBS) solution in intervals. The current was degraded with increased concentration, becoming saturated at a concentration of 0.4 mM. Surprisingly, these results indicate that the enzymatic activity of GOx is preserved after encapsulation in HKUST-1 crystals, which is very promising for the synthesis of bioactive MOF composites. The encapsulation of proteins with different sizes into MOF matrices through our method is general and in significant contrast with the reported infiltration process [57] , [58] , in which the MOF pore sizes must be sufficiently large for protein penetration. However, this method is only available for several specific MOFs with large pores. 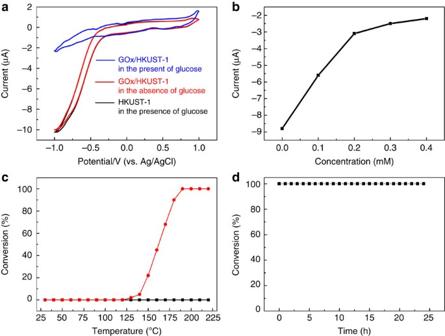Figure 4: Bio-activity and catalytic performance of functional HKUST-1 thin films. The CV performance of (a) HKUST-1 crystals and GOx/HKUST-1 composites in the presence and absence of glucose. (b) The current response of GOx/HKUST-1 to the concentration of glucose by internally adding glucose with a scan rate of 10 mV s−1; CO oxidation catalysed by Au NPs/HKUST-1 composites. (c) Conversion versus temperature (red curve: Au NPs/HKUST-1 composites; black curve: HKUST-1); (d) conversion at 200 °C versus time. The data presented here are the average values recorded from three individual samples, with an average error of approximately 4%. Figure 4: Bio-activity and catalytic performance of functional HKUST-1 thin films. The CV performance of ( a ) HKUST-1 crystals and GOx/HKUST-1 composites in the presence and absence of glucose. ( b ) The current response of GOx/HKUST-1 to the concentration of glucose by internally adding glucose with a scan rate of 10 mV s −1 ; CO oxidation catalysed by Au NPs/HKUST-1 composites. ( c ) Conversion versus temperature (red curve: Au NPs/HKUST-1 composites; black curve: HKUST-1); ( d ) conversion at 200 °C versus time. The data presented here are the average values recorded from three individual samples, with an average error of approximately 4%. Full size image Catalytic performance of Au NP/HKUST-1 composite thin films After encapsulating the functional components into MOFs, synergistic properties are expected. Au NPs have been previously used in the catalytic oxidation of CO [59] , [60] , [61] , [62] . First, the catalytic oxidation of CO through Au NP (20 nm)/HKUST-1 composite thin films was examined. The feed gas flow was composed of 1% CO, 7% O 2 and 92% Ar with a flow rate of 200 s.c.c.m. As shown in Fig. 4c , CO begins to oxidize at 125 °C and is nearly 100% converted at 190 °C. The amount of the Au NP/HKUST-1 composite was 100 mg, with 5 mg Au. Therefore, the catalysis efficiency is 297.62 × 10 −6 mol g Au −1 s −1 at 160 °C, based on 50% conversion. The durability of Au NP/HKUST-1 composites as a catalyst for CO oxidation is shown in Fig. 4d . The horizontal straightness demonstrates the high durability of Au NP/HKUST-1 composite thin films. In contrast to the infiltration encapsulation process, in which particle size is limited by the cavities of the MOF host [27] , in our case, even when the particle size is bigger than the cavities of the host MOFs, their specific functions are reserved due to the highly porous networks of MOFs. The morphology and crystal structure of Au NPs/HKUST-1 are almost unchanged after catalytic reactions ( Supplementary Fig. 13 ), indicating the high stability of the composites. Taking advantage of the size-sieving effect of HKUST-1, Au NP (5 nm)/HKUST-1 composite thin films ( Supplementary Fig. 14 ), both in free-standing form ( Fig. 5a ) and in a catalytic membrane reactor module ( Fig. 5e ), are applied to the hydrogenation of n -hexene and cis -stilbene, respectively. Both olefins exhibit complete conversion with bare Au NPs (5 nm) [27] . However, Au NP (5 nm)/HKUST-1 composite thin films, in both the free-standing form and membrane reactors, demonstrate size-selective catalysis of n -hexene from cis -stilbene because n -hexene is smaller; however, cis -stilbene is larger than the 0.9-nm pore of HKUST-1 (ref. 34 ). In the free-standing form, 50 mg Au NPs (5 nm)/HKUST-1 containing 2.5 mg Au NPs is used. As presented in Fig. 5b , 26.3% catalytic conversion of n -hexene occurs, but no conversion of cis -stilbene was observed at 35 °C for 24 h. This result is likely due to the larger molecular size of cis -stilbene, which diffuses hardly through the pore apertures of the HKUST-1 crystal to reach the catalytic Au NPs. The catalytic performance of n -hexene using the free-standing Au NP (5 nm)/HKUST-1 composite thin film at different temperatures for 2 h is shown in Fig. 5c,d . Upon increasing the temperature, the conversion is significantly enhanced, from 2.3% at 35 °C to 19.3% at 150 °C. Based on both the size-selective catalyst and the continuous and thorough intergrowth of Au NP (5 nm)/HKUST-1 composite thin films, an Au NP/HKUST-1 composite thin film was applied as a catalytic membrane reactor and then was constructed in a stainless steel filter holder with both sealed ends, as shown in Fig. 5e . Maintaining the same catalytic conditions as applied in the free-standing form at 35 °C for 24 h, the final gas compositions in the permeate sides were analysed by gas chromatography. As shown in Fig. 5f , 61.4% n -hexene, 36.3% n -hexane and 2.3% cis -stilbene are present in the permeate. These size-selective catalytic results further confirm that the Au NPs are well encapsulated within the MOF matrices. Therefore, this Au NPs/HKUST-1 thin film can be used for simultaneous gas separation and catalysis. 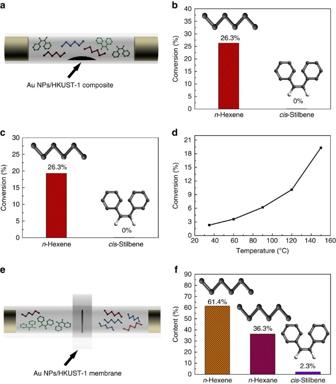Figure 5: Size-selective catalytic performance of Au NP (5 nm)/HKUST-1 thin films. (a) Diagram of the first method using Au/HKUST-1 free-standing samples in the middle of a quartz tube for a liquid-phase hydrogenation experiment; catalytic conversion ofn-hexene andcis-stilbene over Au NP (5 nm)/HKUST-1 powders at (b) 35 °C for 24 h and (c) 150 °C for 2 h; (d) conversion ofn-hexene over Au NP (5 nm)/HKUST-1 free-standing thin films at different temperatures for 2 h. (e) Diagram of the first method using an Au NP/HKUST-1 thin film as a membrane reactor sealed in a stainless steel filter holder for a liquid-phase hydrogenation experiment at 35 °C; (f) after 24 h, the final gas composition of the permeate monitored by GC. The data presented here are the average values recorded from three individual samples, with an average error of approximately 3%. Figure 5: Size-selective catalytic performance of Au NP (5 nm)/HKUST-1 thin films. ( a ) Diagram of the first method using Au/HKUST-1 free-standing samples in the middle of a quartz tube for a liquid-phase hydrogenation experiment; catalytic conversion of n -hexene and cis -stilbene over Au NP (5 nm)/HKUST-1 powders at ( b ) 35 °C for 24 h and ( c ) 150 °C for 2 h; ( d ) conversion of n -hexene over Au NP (5 nm)/HKUST-1 free-standing thin films at different temperatures for 2 h. ( e ) Diagram of the first method using an Au NP/HKUST-1 thin film as a membrane reactor sealed in a stainless steel filter holder for a liquid-phase hydrogenation experiment at 35 °C; ( f ) after 24 h, the final gas composition of the permeate monitored by GC. The data presented here are the average values recorded from three individual samples, with an average error of approximately 3%. Full size image Conductive and flexible SCNT/HKUST-1 composite thin film Notably, in contrast to the insulated and brittle HKUST-1, the SWCNT/HKUST-1 composite thin film ( Fig. 1k,l ) is highly flexible ( Supplementary Fig. 15 and Supplementary Movie 1 ) and highly conductive, with a resistance of only 35 Ω per square, because of the bi-continuous structures of the MOF and SWCNT networks. After incorporating SWCNTs, the composite thin film has a thermal decomposition temperature of 333 °C and Brunauer–Emmett–Teller (BET) surface area of 1,192 m 2 g −1 ( Supplementary Fig. 16 ). The decomposition temperature is slightly higher than that of pure HKUST (330 °C), but the surface area is slightly lower than that of pure HKUST-1 thin films (1,370 m 2 g −1 ) [10] . This difference could be due to the incorporation of SWCNTs, which enhances the thermal stability and reduces the BET surface area of the MOF host. This paper is the first report of flexibly foldable and conductive MOF composite thin films, which may overcome the brittle and insulating drawbacks of MOFs and expand the applications of MOFs for flexible electronic devices. The high aspect ratio, small diameter, high dispersibility and highly positively charged surfaces of MHNs affect the uniform encapsulation of functional components in MOF matrices. As mentioned above, negatively charged ions, particles and carbon nanotubes are easily assembled with positively charged MHNs and form the corresponding uniform composites [49] . The components are not negatively charged, but, if their sizes are larger than the pore size of the mesoporous MHN fibrous thin film, then they can also be incorporated into MHN matrices by filtering a mixture of their suspension with a solution of MHNs ( Supplementary Fig. 1 ). The functional components are firmly confined and uniformly located in MHN networks. In our case, when immersing the functional components/MHNs into an organic linker solution, the outermost surface of the MHN layer rapidly reacts with organic ligands and forms a relatively dense MOF crystal layer ( Supplementary Fig. 17a ). This layer could prevent the escape of functional components and make the growth proceed from the outer side to the inner side of the composite MHN thin film by the gradual conversion of MHNs to MOFs ( Supplementary Fig. 17 ). During this process, the pre-embedded functional components are confined and have no opportunity for significant movement because they are surrounded by MOF crystals. Of course, the balance between the dissolution rate of MHNs and coordination formation of MOFs is crucial for the formation of well-defined component-encapsulated MOF composite thin films [43] . In our case, because of their very positively charged surfaces, MHNs are more active and ready for coordination with organic linkers. Therefore, the coordination rate should be larger than the dissolution rate, resulting in continuous and uniform composite thin films. The entire encapsulation and growth process of composite MOF films are illustrated in Supplementary Fig. 18 . However, the encapsulation of large particles may lead to re-adjustments of the MOF local structure and/or defects, which are not easily detected by XRD or even electron microscopic techniques. The impact of local structure and defects on MOF properties remains unclear and requires further investigation. This method is clearly quite powerful and can successfully encapsulate various types of functional components within MOF thin films at room temperature within 1–2 h. MHNs not only serve as a metal source but also assist the assembly of functional components embedded into precursor networks, which is critical for the preparation of uniform functional component-encapsulated MOF composite thin films. In addition, because the process occurs at room temperature and does not generate acidic by-products, dissociation and degradation of the encapsulated functional agents are prevented. Therefore, bio-active protein-encapsulated MOF thin films are realized and could be desirable for bio-related applications. Thin films with new synergistic properties should be expected by combining the properties of the functional agents and the MOF hosts, and there is promise for thin film-related devices, including catalytic membrane reactors and conductive and flexible electronic devices. Experimental materials Copper nitrate (Cu(NO 3 ) 2 ·3H 2 O), zinc nitrate (Zn(NO 3 ) 2 ·6H 2 O) and 2-aminoethanol (NH 2 –CH 2 CH 2 OH) were purchased from Acros Chemicals. Trimesic acid (H 3 BTC), 1, 4-benzenedicarboxylic acid (H 2 BDC), ferritin (from equine spleen) and GOx (from Aspergillus niger ) were purchased from Sigma-Aldrich. Sodium citrate was purchased from Alfa Aesar. Au NPs (5 nm) were purchased from BBInternational (0.5 mg ml −1 ). HAuCl 4 ·4H 2 O was purchased from Wako Pure Chemical Industries, Ltd. A nitric acid-oxidized SWCNT aqueous dispersion (2 mg ml −1 ) was purchased from Nanjing XFNANO Materials Tech Co., Ltd. PS spheres were purchased from SPI Supplies. NaAuCl 4 was purchased from J&K Chemical. The supports were AAO membranes (Whatman Anopore) with an average pore size of ca 200 nm and porosity of 50%. PS spheres were purchased from SPI on the order of 10 12 –10 14 U ml −1 . Ultrapure water (18.2 MΩ) produced by a Millipore direct-Q system (Millipore) was used throughout the experiments. Preparation of CHNs and ZHNs CHNs were synthesized by rapidly mixing equal volumes of 4 mM copper nitrate solution and 1.4 mM aminoethanol solution at room temperature and ageing for 2 days. ZHNs were synthesized by rapidly mixing 4 mM zinc nitrate solution with 2.0 mM aminoethanol at room temperature and ageing for 30 min (refs 10 , 49 ). Synthesis of Au NPs colloids Citrate-stabilized nanoparticles (20 nm diameter) were prepared using a modification of Frens’ method [63] . All glassware used in the following procedure was cleaned in a bath of freshly prepared 3:1 (HNO 3 :HCl) solution, rinsed thoroughly in water and dried in air. Typically, 4 ml of 38.8 mM sodium citrate was rapidly injected into 50 ml of a vigorously boiling 1 mM HAuCl 4 aqueous solution. The mixed solution was boiled for 10 min and further stirred for 15 min. The resulting solution was cooled to room temperature, filtered and stored in the refrigerator (4 °C). The size and morphology of the prepared AuNPs were characterized by TEM. The concentration of 20 nm Au NPs was calculated to be nearly 0.44 mg ml −1 . Preparation of [AuCl 4 ] − /HKUST-1 composite thin films First, 0.1 ml of 10 mM NaAuCl 4 (pH=7) was mixed with 30 ml of CHN solution and stirred for approximately 5 min. After filtering the mixture solution on an AAO membrane, a [AuCl 4 ] − /CHN thin film was obtained. The obtained film was reacted with 10 ml of a 5 mM H 3 BTC ethanol/water solution with a volume ratio of 1:1 at room temperature. Typically, after 1 h, a [AuCl 4 ] − /HKUST-1 composite thin film was formed. Preparation of Au NP (20 nm)/HKUST-1 composite thin film A 0.5-ml portion of the prepared 20 nm Au NPs colloids was mixed with 30 ml of CHN solution and stirred for approximately 5 min. After filtering the mixture solution on an AAO membrane, an Au NP/CHN thin film was obtained and reacted with 10 ml of a 5 mM H 3 BTC ethanol/water solution with a volume ratio of 1:1 at room temperature for 1 h. An Au NP (20 nm)/HKUST-1 composite thin film was thus formed. Preparation of Au NP (5 nm)/HKUST-1 composite thin film A 0.5-ml portion of the purchased 5 nm Au NPs colloids was mixed with 30 ml of CHN solution and stirred for approximately 5 min. After filtering the mixture solution on an AAO membrane, an Au NP/CHN thin film was obtained and reacted with 10 ml of a 5 mM H 3 BTC ethanol/water solution with a volume ratio of 1:1 at room temperature for 1 h. An Au NP (5 nm)/HKUST-1 composite thin film was thus formed. Preparation of Au NP/MOF-5 composite thin film A 0.5-ml portion of the prepared 20-nm Au NPs colloids was mixed with 30 ml of ZHN solution and stirred for approximately 5 min. After filtering the mixture solution on an AAO membrane, an Au NP/ZHN thin film was obtained and reacted with 10 ml of 10 mM H 2 BDC DMF solution at room temperature for 1 h. An Au NP (20 nm)/MOF-5 composite thin film was thus formed. Preparation of ferritin/HKUST-1 composite thin film Typically, 0.1 ml of 5 mg ml −1 ferritin was mixed with 30 ml of CHN solution and filtered on an AAO membrane, then reacted with 10 ml of 5 mM H 3 BTC ethanol/water solution with a volume ratio of 1:1 at room temperature for 2 h. Preparation of GOx/HKUST-1 composite thin film A 0.1-ml portion of 5 mg ml −1 GOx was mixed with 30 ml of CHN solution and stirred for approximately 5 min. After filtering the mixture solution on an AAO membrane, a GOx/CHN thin film was obtained, which was then peeled from the AAO support and immersed in 10 ml of 5 mM H 3 BTC ethanol/water solution with a volume ratio of 1:1 at room temperature. After 2 h, a free-standing GOx/HKUST-1 composite thin film was obtained. Preparation of PS/HKUST-1 composites A 0.5-μl portion of a stock suspension of PS spheres with sizes of 620 and 1,000 nm was mixed with 30 ml of CHN solution and stirred for approximately 5 min, respectively. After filtering the mixture solutions on AAO membranes and immersing in 10 ml of 5 mM H 3 BTC ethanol/water solution with a volume ratio of 1:1 for 1 h, PS/HKUST-1 composite thin films were obtained. Preparation of SWCNT/HKUST-1 composite thin film First, SWCNT/CHN thin films were prepared by filtering a mixture of 0.5 ml of 1 mg ml −1 SWCNT solution and 30 ml of CHN solution on an AAO membrane. Then, SWCNT/HKUST-1 composites were formed by immersing the prepared SWCNT/CHN composite film into 10 ml of 5 mM H 3 BTC ethanol/water solution with a volume ratio of 1:1 at room temperature for 1 h. Preparation of HKUST-1/PS/HKUST-1 composites First, 15 ml of CHNs was filtered on an AAO membrane, then a PS layer was formed on its surface by filtering 10 ml of a diluted suspension of 620-nm PS spheres (from 0.5 μl of stock PS colloids). Subsequently, another 15 ml of CHN solution was filtered on the surface of the PS layer. Finally, the CHN/PS/CHN composite thin film was immersed into 10 ml of 5 mM H 3 BTC ethanol/water solution with a volume ratio of 1:1 at room temperature for 1 h and converted to a HKUST-1/PS/HKUST-1 sandwich composite film. Preparation of HKUST-1/SWCNT/HKUST-1 sandwich thin film Similar to the procedure applied for the synthesis of HKUST-1/PS/HKUST-1 sandwich thin films, first, a CHN/SWCNT/CHN sandwich thin film was prepared by alternately filtering 15 ml of CHN solution, 0.05 ml of 1 mg ml −1 SWCNT solution and 15 ml of CHN solution on a porous substrate. Then, the preformed composite thin film was immersed in 10 ml of 5 mM H 3 BTC ethanol/water solution with a volume ratio of 1:1 and continued reacting at room temperature for 1 h. Preparation of Au NPs and ferritin co-encapsulated HKUST-1 composite thin film Typically, 0.1 ml of 5 mg ml −1 ferritin and 0.5 ml of the prepared 20 nm Au NPs colloids were mixed with 30 ml of CHN solution and filtered on an AAO membrane, then reacted with 10 ml of 5 mM H 3 BTC ethanol/water solution with a volume ratio of 1:1 at room temperature for 2 h. Then, Au NPs and ferritin co-encapsulated HKUST-1 composite thin films were formed. Characterization The phases of the as-prepared products were characterized by XRD at room temperature using an X’Pert PRO (PANalytical) instrument with Cu Kα radiation. The morphologies and structures were characterized by SEM (Hitachi, S-4800) with EDS and TEM (Tecnai, G2 F20 S-TWIN). SEM observations were conducted after coating a thin platinum layer with a Hitachi e-1030 ion sputter at a pressure of 10 Pa and current density of 10 mA. Enzymatic activity of GOx/HKUST-1 composite thin film A GCE was cleaned by polishing with alumina powders and then rinsed with ethanol and deionized water successively. An approximately 2-mm piece of GOx/HKUST-1 composite thin film was loaded on the GCE surface and fixed by dropping 5 μl of chitosan solution (0.5 wt.% with 2% acetic acid) and drying for 2 h. The GOx/HKUST-1 electrode was then rinsed with PBS to remove loosely adsorbed GOx and stored at 4 °C. The electrochemical bioactivity of GOx/HKUST-1 was examined by CV conducted in PBS solution in the presence of glucose. A platinum counter electrode and an Ag/AgCl reference electrode were used. All electrochemical experiments were performed with a WPG100e electrochemical workstation. CO catalytic oxidation of Au NP/HKUST-1 composite thin film Approximately 100 mg of Au NP (20 nm)/HKUST-1 composite thin films with approximately 5 mg of Au nanoparticles were loaded in the middle of a quartz tube (diameter 8 mm) that was mounted on a tube furnace. A gas flow (200 s.c.c.m.) mixture of CO (1%), O 2 (7%) and He (92%) was used. The composition of the effluent gas was analysed using a gas chromatograph (GC 9790, Zhejiang Fuli Analysis Equipment Company). Au (5 nm)/HKUST-1 composite films for catalytic hydrogenation (i) The hydrogenation of n -hexene and cis -stilbene was carried out in a quartz tube with diameter of 8 mm under a static hydrogen atmosphere (1 bar). An Au NP (5 nm)/HKUST-1 free-standing composite thin film (50 mg with 5 mg Au NPs) was loaded in the middle of the quartz tube. n -Hexene (0.5 ml) or cis -stilbene (0.5 ml) was then introduced into the quartz tube. After sealing both ends of the tube, hydrogen was used to purge two or three times subsequently, the reaction was carried out at a pre-set temperature for a certain amount of time. After the reaction, the products were analysed by GC. (ii) The Au NP (5 nm)/HKUST-1 composite thin film (50 mg) with 2.5 mg Au NPs (5 nm) on AAO was mounted on a stainless steel filter system (Millipore, XX4502500, 25 mm, max inlet pressure 345 bar). Then, n -hexene (0.5 ml) and cis -stilbene (0.5 ml) were introduced together on one side of the membrane. After sealing both ends of the system, hydrogen was used to purge two or three times subsequently, the reaction proceeded at a pre-set temperature for a certain amount of time. After the reaction, the products on the permeate side were analysed using GC. How to cite this article : Mao, Y. et al. General incorporation of diverse components inside metal-organic framework thin films at room temperature. Nat. Commun. 5:5532 doi: 10.1038/ncomms6532 (2014).